Efficient room-temperature nuclear spin hyperpolarization of a defect atom in a semiconductor Nuclear spin hyperpolarization is essential to future solid-state quantum computation using nuclear spin qubits and in highly sensitive magnetic resonance imaging. Though efficient dynamic nuclear polarization in semiconductors has been demonstrated at low temperatures for decades, its realization at room temperature is largely lacking. Here we demonstrate that a combined effect of efficient spin-dependent recombination and hyperfine coupling can facilitate strong dynamic nuclear polarization of a defect atom in a semiconductor at room temperature. We provide direct evidence that a sizeable nuclear field (~150 Gauss) and nuclear spin polarization (~15%) sensed by conduction electrons in GaNAs originates from dynamic nuclear polarization of a Ga interstitial defect. We further show that the dynamic nuclear polarization process is remarkably fast and is completed in <5 μs at room temperature. The proposed new concept could pave a way to overcome a major obstacle in achieving strong dynamic nuclear polarization at room temperature, desirable for practical device applications. Spintronics is a new paradigm for future electronics and photonics, which explores the spin degree of freedom instead of or in addition to electron charge [1] , [2] , [3] , [4] , [5] , [6] , [7] . Among many formidable challenges, efficient nuclear spin hyperpolarization and manipulation at room temperature (RT) are essential to the success of future solid-state quantum computation using nuclear spin qubits [8] , [9] , [10] , [11] , [12] , [13] , [14] , [15] , [16] , as well as in highly sensitive magnetic resonance imaging (MRI) [17] , [18] . The most common approach employed so far in achieving nuclear spin hyperpolarization is based on dynamic nuclear polarization (DNP). By strongly deviating electron spin distribution from thermal equilibrium by an external means, subsequent electron spin redistribution towards thermal equilibrium can trigger electron–nuclear (e–n) spin transfer leading to nuclear spin imbalance that can be several orders of magnitude larger than that in thermal equilibrium. When microwave saturation [19] or optical electronic saturation [20] , [21] that attempts to equalize populations between Zeeman-split electron spin sublevels is employed as an external driving force, the enhancement in nuclear spin polarization ( P N ) relies on a large electron spin polarization degree in thermal equilibrium. Therefore, it is only restricted to very low temperatures and requires a strong external magnetic field. An alternative approach by optical pumping, on the other hand, is free from these restrictions because a large electron spin imbalance can now be generated by optical pumping and no spin imbalance is required in thermal equilibrium. As a result, DNP by optical pumping should in principle be capable of generating strong P N even at RT. This approach is especially attractive for semiconductors, where the selection rules for the band-to-band optical transitions allow selective spin generation of conduction-band electrons by circularly polarized light –an approach commonly referred to as optical orientation [22] . Though efficient DNP by optical orientation has indeed been demonstrated at low temperatures for decades [22] , [23] , its realization at RT is practically non-existing. The main problem lies on rapidly accelerated spin relaxation of conduction-band electrons at RT known in semiconductors [2] , [22] , which diminishes the effect of optical spin orientation. This leads to weak spin polarization (close to the thermal equilibrium value) for both conduction-band electrons and electrons localized at defect centres that are coupled to local nuclear spins, making DNP improbable. The only exception when a combination of optical and microwave pumping has made RT nuclear spin polarization possible is the recent demonstration of a quantum register based on 13 C nuclear spins neighbouring the nitrogen-vacancy centre in diamond [12] . In this case, the problem was circumvented by directly generating electron spin polarization at the defect centre via resonant optical excitation of the localized states without involvement of conduction-band electrons [12] and thereby removing the restriction imposed by strong conduction-band electron spin relaxation. Further extending to solids in general, perhaps the only other exceptional case when RT DNP was possible is the polarization transfer from the photo-excited triplet state of the guest pentacene molecule to the protons of the naphthalene host molecular crystal [24] . A similar approach to the nitrogen-vacancy centre in diamond was used, namely by resonant optical excitation of localized electron spin state. In this work, we seek for an alternative solution by directly tackling the problem of conduction-band electron spin polarization at RT. This approach is attractive as it involves spin-polarized conduction-band electrons that can be generated by optical pumping or electrical spin injection, which paves a way for electrical control of DNP at RT—a desirable property for practical device applications. It also provides a means to polarize nuclear spins of different paramagnetic centres and also host atoms all at once, which is relevant not only to significant enhancement of sensitivity at RT for nuclear MRI but also to initialization of nuclear spin qubits that are not directly accessible by resonant optical excitation. Our approach exploits the recently discovered defect-engineered spin-filtering effect [25] , which has been demonstrated to be capable of generating strong spin polarization of conduction-band electrons in a semiconductor at RT. Strong conduction-band electron spin polarization of >40% can be obtained at RT in Ga(In)NAs by spin-filtering through Ga i interstitial defects [25] , [26] , [27] , [28] , [29] . By taking advantage of the spin-filtering effect and going beyond merely generating conduction-band electron spin polarization that was the focal point of the previous studies [25] , [26] , [27] , [28] , [29] , we shall show in this work that strong and efficient nuclear spin polarization of the core Ga atom of the Ga i defects can be achieved at RT by optical orientation. This represents the first demonstration of DNP of a defect nucleus induced by optical pumping of conduction-band electrons at RT in a semiconductor. Spin-filtering enabled nuclear spin hyperpolarization The principle of the proposed DNP process is schematically shown in Fig. 1 . For simplicity, we take as an example a simple e–n spin system with a single unpaired electron ( S =1/2) localized at a defect and a nuclear spin I =1/2 of the defect atom ( Fig. 1a–d ). Four relative orientations between the electron and nuclear spins are possible, that is, ↑ , ↑ , ↓ and ↓ . Here, the first and second arrows represent electron and nuclear spin orientations, respectively. As described in detail in the Methods section, when the defect-engineered spin-filtering is in action, the four possible spin configurations will follow the paths illustrated by the dashed arrows shown in Fig. 1a–d and will all eventually end up with ↑ as the final and stable spin configuration. In other words, a combined effect of spin-dependent recombination (SDR) and hyperfine (HF) coupling can align both localized electron spin and nuclear spin towards the direction of the conduction-band electron spins generated by the spin-filtering effect, and will lead to strong spin polarization of both electron and nucleus at the defect. It should be pointed out that the principle described above should remain valid even when the conduction-band electrons are not completely spin polarized, though a less efficient DNP process could be expected in such a case. The described physical principle of the DNP process can easily be extended to other more complicated e–n systems, such as that studied in this work with S =1/2 and I =3/2 as illustrated in Fig. 1e . They only differ by the number of steps of the SDR and e–n spin flip-flop process required before complete nuclear spin polarization can be achieved. 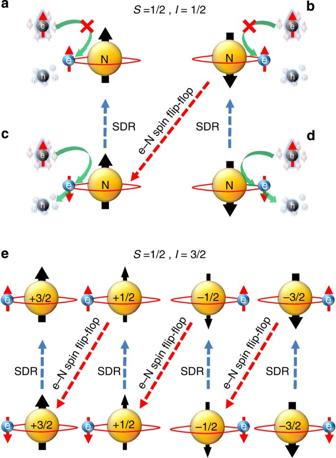Figure 1: Principle of the spin-filtering enabled nuclear spin hyperpolarization at RT and zero field. Four possible relative orientations of an e–n spin system withS=1/2 andI=1/2: (a) ↑, (b) ↑, (c) ↓and (d) ↓. (e) The spin configurations of an e–n spin system withS=1/2 andI=3/2, relevant to the spin-filtering Gaidefects in GaNAs. Strong spin polarization of the free conduction-band electrons is generated by the defect-engineered spin-filtering effect. The flow directions of the spin configurations under the influence of SDR and HF coupling are indicated by the dashed arrows. The yellow and blue balls represent the nucleus and electron of a defect, respectively, with the arrows indicating their spin orientations. The conduction-band electrons and valence-band holes are depicted by the grey balls marked by e and h, respectively. Figure 1: Principle of the spin-filtering enabled nuclear spin hyperpolarization at RT and zero field. Four possible relative orientations of an e–n spin system with S =1/2 and I =1/2: ( a ) ↑ , ( b ) ↑ , ( c ) ↓ and ( d ) ↓ . ( e ) The spin configurations of an e–n spin system with S =1/2 and I =3/2, relevant to the spin-filtering Ga i defects in GaNAs. Strong spin polarization of the free conduction-band electrons is generated by the defect-engineered spin-filtering effect. The flow directions of the spin configurations under the influence of SDR and HF coupling are indicated by the dashed arrows. The yellow and blue balls represent the nucleus and electron of a defect, respectively, with the arrows indicating their spin orientations. The conduction-band electrons and valence-band holes are depicted by the grey balls marked by e and h, respectively. Full size image Optical orientation in a longitudinal magnetic field To detect DNP we employed a commonly used method of optical orientation in an external magnetic field ( B z ) [22] , [23] applied along the direction of optical excitation and detection, as illustrated in Fig. 2a . As schematically shown in Fig. 2b , the application of B z should suppress depolarization of optically generated electron spins S 0 caused by Larmor precession of the electron spins around a randomly fluctuating effective magnetic field ( B F ), leading to an increase in electron spin projection < S z > along the field and thus spin polarization with increasing field strength [22] , [23] , [29] . A nuclear field B N generated by DNP along the direction of the optical spin orientation can either add to or compensate the external field, depending on its relative orientation with B z (that is, parallel or antiparallel). The minimum electron spin polarization should, therefore, occur at a finite external magnetic field, when the total effective longitudinal field is zero, that is, B z +< B N >=0 or B z =−< B N >, which corresponds to an Overhauser shift [19] . Here, < B N > denotes an average local nuclear field within the volume of a sample that is subject to optical excitation. As spin polarization and total concentration of conduction-band electrons are inter-connected by the defect-engineered spin-filtering effect [25] , [26] , [27] , [28] , [29] , see Supplementary Fig. S1 , < B N > can be conveniently measured by monitoring either circular polarization or total intensity of the band-to-band photoluminescence as a function of B z . Typical experimental results obtained at RT from a GaNAs epilayer are shown in Fig. 2c , by monitoring the difference between the photoluminescence intensities under circular ( σ + or σ − ) and linear ( σ x ) excitation that are modulated at 135 Hz as illustrated in Fig. 2a . This modulation scheme increases the reliability of the results, because it directly measures the contrast between the cases with and without optical generation of electron spin polarization. An Overhauser shift of about 100 Gauss is clearly seen under optical pumping at 150 mW, yielding < B N >=−100 Gauss under σ + excitation and < B N >=+100 Gauss under σ − excitation. The observed change in the sign of < B N > is consistent with the assumption that DNP is caused by the spin-polarized conduction-band electrons that change their spin orientation when the helicity of circularly polarized excitation light is switched between σ + and σ − . The Overhauser shift is found to decrease with decreasing excitation power, as shown in Fig. 2c , which is largely expected for a dynamic process such as DNP. The Overhauser shift and its dependence on optical pumping power can be observed in all studied GaNAs samples as long as the defect-engineered spin-filtering effect is active. The exact < B N > value varies between the samples, however, critically depending on the N composition of the alloys and post-growth treatments [25] , [30] . As examples, the |< B N >| values from two GaNAs samples of different N compositions are shown in Fig. 2d as a function of optical pumping power. 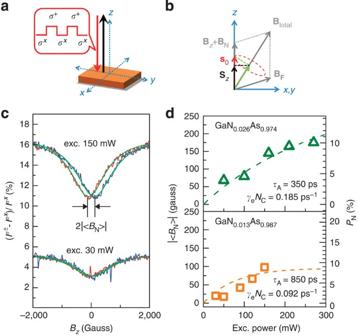Figure 2: Observation of overhauser shift at RT. (a) A schematic picture of the experimental configuration, where the optical excitation and photoluminescence detection are indicated by the red and black arrows, respectively. The modulation scheme of the excitation light, at a modulation frequency of 135 Hz, is also shown. (b) A pseudospin description of the optically pumped electron spinS0and its projectionSzunder a combined effect of a fluctuating effective magnetic fieldBF, a longitudinal external magnetic fieldBzand an optically induced nuclear fieldBN. (c) The total intensity of the band-to-band photoluminescence as a function ofBzunderσ+(the blue curves) orσ−(the red curves) excitation (denoted by), with respect to that under linear (σx) excitation (), obtained at RT from GaN0.013As0.987after rapid thermal annealing treatment. The excitation wavelength was 930 nm, and excitation power levels were 150 and 30 mW. The solid green lines are Lorentzian fits of the experimental curves. (d) The absolute values of an average nuclear field () and the correspondingPNof the Gaidefects, as a function of optical pumping power for the specified GaNAs epilayers. The open symbols represent the experimental data. The dashed lines are calculated values obtained from a rate equation analysis, with the specified key fitting parameters. Other fitting parameters areT1SC=5 ns andτN=10 ns. The deduced difference in the e–n spin flip-flop timeτAbetween the two samples is consistent with what is expected from the difference in the HF coupling constantAof the Gaidefects present in these samples. Figure 2: Observation of overhauser shift at RT. ( a ) A schematic picture of the experimental configuration, where the optical excitation and photoluminescence detection are indicated by the red and black arrows, respectively. The modulation scheme of the excitation light, at a modulation frequency of 135 Hz, is also shown. ( b ) A pseudospin description of the optically pumped electron spin S 0 and its projection S z under a combined effect of a fluctuating effective magnetic field B F , a longitudinal external magnetic field B z and an optically induced nuclear field B N . ( c ) The total intensity of the band-to-band photoluminescence as a function of B z under σ + (the blue curves) or σ − (the red curves) excitation (denoted by ), with respect to that under linear ( σ x ) excitation ( ), obtained at RT from GaN 0.013 As 0.987 after rapid thermal annealing treatment. The excitation wavelength was 930 nm, and excitation power levels were 150 and 30 mW. The solid green lines are Lorentzian fits of the experimental curves. ( d ) The absolute values of an average nuclear field ( ) and the corresponding P N of the Ga i defects, as a function of optical pumping power for the specified GaNAs epilayers. The open symbols represent the experimental data. The dashed lines are calculated values obtained from a rate equation analysis, with the specified key fitting parameters. Other fitting parameters are T 1SC =5 ns and τ N =10 ns. The deduced difference in the e–n spin flip-flop time τ A between the two samples is consistent with what is expected from the difference in the HF coupling constant A of the Ga i defects present in these samples. Full size image To obtain a quantitative understanding of the relevant processes leading to the observed DNP, we have carried out a detailed analysis of the DNP process with the aid of coupled rate equations including all relevant e–n spin sublevels. By self-consistently and simultaneously fitting both the experimentally measured conduction-band electron spin polarization and the nuclear field with the same set of parameters, we are able to obtain a good agreement between the simulated and measured results of |< B N >| and P N as a function of optical pumping power as shown in Fig. 2d . A detailed description of the rate equation analysis is given in the Supplementary Methods . The higher |< B N >| value observed in the GaN 0.026 As 0.974 epilayer as compared with the GaN 0.013 As 0.987 epilayer can be explained by a stronger HF coupling and a high concentration of the spin-filtering Ga i defects in the former, as reflected by the deduced fitting parameters given in Fig. 2d . The stronger HF coupling should lead to a shorter e–n spin flip-flop time τ A , based on 1/ τ A A 2 according to the Fermi’s golden rule. Higher concentrations of the Ga i defects are expected in GaN 0.026 As 0.974 with a higher N composition, because the formation of the Ga i defects is known to be facilitated by incorporation of N [25] , [30] . This should increase the efficiency of the spin-filtering effect [25] , leading to stronger electron spin polarization and thus DNP. Optically detected magnetic resonance To identify the microscopic origin of the observed Overhauser shift and the associated nuclear field, we resorted to the optically detected magnetic resonance (ODMR) technique (for a review on ODMR see ref. 31 ). Representative ODMR spectra under optical pumping obtained at 2 K are displayed in Fig. 3b . They are characteristic for a Ga i defect with an unpaired electron spin ( S =1/2), of which the s-type wavefunction is centred at the Ga i atom [25] . The energy levels of the electron and nuclear spin states for the studied Ga i defect, as well as the exact field positions of the ODMR lines, can be calculated by an analysis of the corresponding spin Hamiltonian (see the Methods section). They are shown in Fig. 3a for each of the 69 Ga and 71 Ga isotopes. 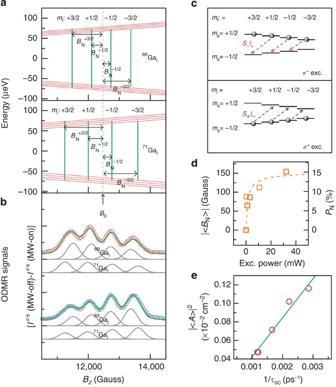Figure 3: Direct evidence for nuclear spin polarization of the defect atom. (a) The calculated energy levels of the electron and nuclear spin states of the Gaidefect for both Ga isotopes. All simulations and calculations were obtained by the spin Hamiltonian with the parameters for the Gai-D defect. The dashed vertical line marks the expected ODMR field position without considering the HF interaction. The solid vertical lines indicate the ODMR fields for the four nuclear spin orientations, by including the HF interaction. The nuclear field () induced by the central Ga nucleus of the defect with the givenare indicated by the horizontal solid arrows. (b) ODMR spectra obtained from GaN0.0036As0.9964underσ+(the blue open circles) andσ−(the red open circles) excitation at 32 mW and 2 K, with a microwave frequency of 35.07 GHz. The solid curves are the simulated ODMR spectra of the Gai-D defect by including contributions from both Ga isotopes (denoted by the grey lines). (c) A schematic diagram of the electron and nuclear spin sublevels in a fixedBz, and the physical mechanism for the observed DNP. The HF-induced e–n spin flip-flops are indicated by the dashed arrows, which point to opposite directions underσ+andσ−excitation leading to a nuclear field of opposite sign. (d) The absolute value of an average nuclear fieldarising from the DNP of the Ga atom of the Gai-D defect as a function of optical pumping power, determined from the ODMR data. The dashed line is obtained from a rate equation analysis, with the key fitting parametersτA=960 ps andγeNc=0.0012, ps−1. (e) Correlation between the electron spin lifetimeτSCmeasured at RT from Hanle effect experiments and the average HF coupling constant <A> of the Gaidefects in different samples determined from the ODMR studies. The open symbols represent the experimental data, of which each data point is taken from a different sample. The solid line is the fitting curve following the relation 1/τSC2. Figure 3: Direct evidence for nuclear spin polarization of the defect atom. ( a ) The calculated energy levels of the electron and nuclear spin states of the Ga i defect for both Ga isotopes. All simulations and calculations were obtained by the spin Hamiltonian with the parameters for the Ga i -D defect. The dashed vertical line marks the expected ODMR field position without considering the HF interaction. The solid vertical lines indicate the ODMR fields for the four nuclear spin orientations, by including the HF interaction. The nuclear field ( ) induced by the central Ga nucleus of the defect with the given are indicated by the horizontal solid arrows. ( b ) ODMR spectra obtained from GaN 0.0036 As 0.9964 under σ + (the blue open circles) and σ − (the red open circles) excitation at 32 mW and 2 K, with a microwave frequency of 35.07 GHz. The solid curves are the simulated ODMR spectra of the Ga i -D defect by including contributions from both Ga isotopes (denoted by the grey lines). ( c ) A schematic diagram of the electron and nuclear spin sublevels in a fixed B z , and the physical mechanism for the observed DNP. The HF-induced e–n spin flip-flops are indicated by the dashed arrows, which point to opposite directions under σ + and σ − excitation leading to a nuclear field of opposite sign. ( d ) The absolute value of an average nuclear field arising from the DNP of the Ga atom of the Ga i -D defect as a function of optical pumping power, determined from the ODMR data. The dashed line is obtained from a rate equation analysis, with the key fitting parameters τ A =960 ps and γ e N c =0.0012, ps −1 . ( e ) Correlation between the electron spin lifetime τ SC measured at RT from Hanle effect experiments and the average HF coupling constant < A > of the Ga i defects in different samples determined from the ODMR studies. The open symbols represent the experimental data, of which each data point is taken from a different sample. The solid line is the fitting curve following the relation 1/ τ SC 2 . Full size image Following the ODMR selection rules, that is, and , four ODMR transitions are expected for each isotope that fulfill the condition . ( h is the Planck constant and ν the microwave frequency used in the ODMR experiment. m s and m I are the projections of the electron and nuclear spin angular momenta along the z direction.) is the local nuclear (Overhauser) field introduced by the Ga nucleus with the nuclear spin orientation , where if the non-secular HF interaction is neglected. Thus, each ODMR transition at the field monitors a specific nuclear spin orientation as indicated on the top of Fig. 3a . It shifts from the ODMR field without the HF coupling , marked by the dashed vertical line in Fig. 3a , by . As the magnetic-dipole transition probability and lifetimes of the spin sublevels are expected to remain the same over the field range of the ODMR transitions, the intensity of each ODMR line provides a direct measure of the relative concentration of the defect in a given nuclear spin state and isotope. Judging from the relative intensity of the low-field and high-field ODMR lines, see Fig. 3b , it is apparent that optical pumping indeed leads to nuclear spin polarization, with σ + and σ − light favoring the spin-down and spin-up nuclear spin orientation, respectively. This can be explained by e–n spin flip-flops driven by the non-secular HF interaction, as schematically illustrated in Fig. 3c . Under σ − excitation, spin-up conduction-band and defect electrons are preferably generated leading to a large deviation of the electron distribution from thermal equilibrium. This will trigger the e–n spin flip-flops governed by the operator , in favour of a positive . The situation should be reversed under σ + excitation. In order to provide a direct comparison with the nuclear fields deduced from the band-to-band photoluminescence under optical orientation in B z shown in Fig. 2 , an average nuclear field from all four nuclear spin orientations and two Ga isotopes of the Ga i defect should be determined from the ODMR data. This can be done by the following relation Similarly, P N of the Ga i defect can be estimated by Here, denotes the intensity of the ODMR line involving . It can be obtained by deconvoluting the experimental ODMR spectra based on a best fit of the spin Hamiltonian including both Ga isotopes. The simulated ODMR lines for each isotope are shown by the grey lines in Fig. 3b . The simulated ODMR spectra including both isotopes are also shown by the green curves, which are in excellent agreement with the experimental data and thus justify the deduced . and P N values, determined by equations 1 and 2 from the ODMR results and averaged between σ + and σ − excitation, are shown by the open squares in Fig. 3d as a function of optical pumping power. A clear trend of an increasing nuclear field (up to 150 Gauss) and P N (up to 15%) with increasing optical pumping power can be observed from the ODMR data. The maximum local nuclear field attainable for the Ga i defect occurs when (corresponding to the cases when P N =±100%), that is, that is 927 G (1178 G) for the 69 Ga ( 71 Ga) isotope of the concerned Ga i defect. These experimental results can be well accounted for by the rate equation analysis as described in the Supplementary Methods , see the dashed line in Fig. 3d for the simulated results. The similarity in the magnitude and excitation power dependence between the Overhauser shift detected in optical orientation experiments and the local nuclear field of the Ga i defects determined by ODMR is indicative of a close link between the two. This is further supported by the fact that the same rate equation analysis yield good agreement with both optical orientation and ODMR results. In the Discussion section below, we will provide further evidence that the nuclear spin polarization of the central Ga atom at the core of the Ga i defects is the origin of the observed DNP at RT. In principle, there could be several possible mechanisms for the Overhauser field observed in the optical orientation experiments shown in Fig. 2 . One possibility could be due to spin-polarized electrons localized at the defects, which could create an effective magnetic field acting on conduction-band electrons. We can rule out this possibility here based on the following facts. First of all, the strength of a direct spin–spin interaction between the conduction-band and defect electrons should depend on their wavefunction overlap, which can be enhanced by increasing the number of conduction-band electrons. The observed trend of slow-down and eventual saturation of the Overhauser field with increasing excitation power, as partly shown in Figs 2d and 3d , seems to be inconsistent with the linear dependence expected for the spin–spin interaction. Secondly, if there existed a sizeable spin–spin interaction between the conduction-band and defect electron, the defect electron could in turn experience a corresponding effective magnetic field imposed by the spin-polarized conduction-band electrons. This would result in noticeable perturbation of the energies of the electron and nuclear spin sublevels of the defect, leading to changes in the ODMR field positions of the defect at different optical pumping power. This was against our experimental finding as the ODMR fields remain the same, except for a change in the relative intensities of the four HF-split lines due to nuclear spin polarization. We can also safely rule out a possible, sizeable contribution to the observed Overhauser field from nuclear spin polarization of the ligand atoms or host atoms surrounding the defects, because it would otherwise cause a noticeable shift of the ODMR lines that was not observed in our experiments. This leaves DNP of the central Ga atom of the Ga i defects as the main source of the Overhauser field observed at RT. Though the Overhauser field cannot be determined at RT simultaneously by optical polarization and ODMR, due to the instrumental limitation for the latter as described in the Methods section, this conclusion is supported by the following experimental findings. Firstly, the Ga i defects have been identified as the source of the defect-engineered spin-filtering/amplification effect that has led to strong spin polarization of conduction-band electrons [25] , [32] . From Hanle experiments, conduction-band electron spin polarization at RT is nearly entirely governed by the spin polarization of the electron localized at the defect [32] , [33] . It is, therefore, natural to expect that even a slight alternation in the spin polarization of the defect electron by the nuclear field induced by the DNP of the Ga i defect can result in a sizeable change in conduction-band electron spin polarization. Secondly, a close and direct correlation was found between defect electron spin relaxation time τ SC obtained at RT from Hanle measurements and the average HF coupling constant < A > of the Ga i defects determined from ODMR, as shown in Fig. 3e . The deduced relation 1/ τ SC 2 can only be explained if τ SC is dominated by the e–n spin flip-flop time τ A , because only τ A obeys the relation 1/ τ A A 2 according to the Fermi’s golden rule. These results also show that τ A is fast (in the order of hundreds of ps), setting the ultimate speed of the DNP process. Another direct correlation between the Overhauser field and the Ga i defects can be found by the strength of B z required to overcome the depolarization caused by B F , which is very close to what is expected if B F originates from the randomly fluctuating nuclear field of the central Ga atom of the Ga i defects (that is, B F ~ ). We should point out that the nuclear field induced by the nuclear spin polarization of the Ga atom at the defect core is directly experienced by the electron localized at the defect. The conduction-band electrons only indirectly sense it as the efficiency of the spin-filtering effect via the defect is determined by the defect electron spin polarization, which is the weakest when the external magnetic field cancels out the nuclear field. Therefore, this work has also provided an unusual and attractive approach where conduction-band electrons can be employed to sense a local nuclear field without actually experiencing it directly, such that the electronic structure and spin configuration of the conduction-band electrons remain intact. The speed of DNP is an important factor for practical applications as it determines the initialization speed of nuclear spin qubits or the rate of nuclear spin hyperpolarization for MRI. To evaluate the speed of the studied DNP of the defect nucleus, we performed optical orientation studies at RT by applying alternating circularly polarized light between σ + and σ − . If the DNP process cannot follow the alternating speed of the circularly polarized light, no nuclear field is expected to build-up. The results at a modulation frequency of 10 kHz are shown in Fig. 4a , recorded by monitoring the total intensity of the band-to-band photoluminescence as a function of B z and time over which the excitation polarization alternates. The Overhauser shift is clearly visible, and switches its direction whenever the excitation light switches polarization. Cross-section plots of Fig. 4a at two given times (41 μs and 91 μs) corresponding to pure σ + and σ − excitation are displayed by the blue and red open circles in Fig. 4b , respectively. They clearly confirm a sizeable Overhauser shift of about 150 Gauss in both cases. The result is similar to what was observed under the continuous-wave σ + or σ − excitation shown in Fig. 2c . To further verify the fast response of the observed DNP, we studied the differential photoluminescence intensity under alternating σ + and σ − excitation by the lock-in technique. The experimental curve at a modulation frequency of 10 kHz is displayed by the upper curve in Fig. 4c , which is equivalent to a subtraction between the two curves in Fig. 4b . The observed derivative-like response is a result of the opposite Overhauser shifts occurring under σ + and σ − excitation. A similar result is also obtained under alternating circularly polarized light excitation at 100 kHz, shown by the lower curve in Fig. 4c . This must mean that the DNP process of the defect atom is remarkably fast, with a build-up time of <5 μs—shorter than the response time of our instruments. This finding is in good agreement with the short τ A determined from the RT Hanle measurements ( Fig. 3e ) and the rate equation analysis ( Figs 2d and 3d ). 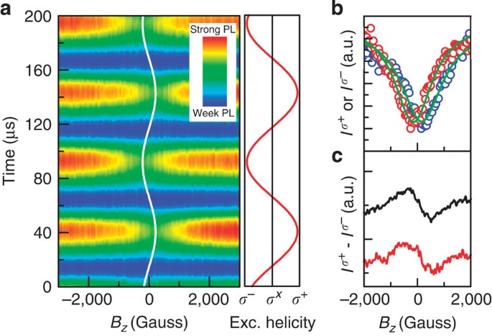Figure 4: Experimental proof for fast DNP. (a) Left panel: A two-dimensional plot of the total photoluminescence intensity of the band-to-band optical transition under alternatingσ+andσ−excitation as a function of time andBz, obtained at RT from GaN0.026As0.974. The contrast from blue to red colour corresponds to weak to strong photoluminescence intensity. The white line is a guide to the eye, signifying the Overhauser shift. Right panel: The helicity of the excitation light as a function of time. (b) The horizontal cross-sectional plots ofaat 41 (the blue open circles) and 91 μs (the red open circles), which correspond to the photoluminescence intensity obtained under pureσ+andσ−excitation, respectively. The solid lines are Lorentzian fits of the experimental curves. (c) Differential photoluminescence intensity betweenσ+andσ−excitation modulated at 10 (the black curve) and 100 kHz (the red curve), obtained by the locking-in technique in phase withσ+excitation. a.u., arbitrary unit. Figure 4: Experimental proof for fast DNP. ( a ) Left panel: A two-dimensional plot of the total photoluminescence intensity of the band-to-band optical transition under alternating σ + and σ − excitation as a function of time and B z , obtained at RT from GaN 0.026 As 0.974 . The contrast from blue to red colour corresponds to weak to strong photoluminescence intensity. The white line is a guide to the eye, signifying the Overhauser shift. Right panel: The helicity of the excitation light as a function of time. ( b ) The horizontal cross-sectional plots of a at 41 (the blue open circles) and 91 μs (the red open circles), which correspond to the photoluminescence intensity obtained under pure σ + and σ − excitation, respectively. The solid lines are Lorentzian fits of the experimental curves. ( c ) Differential photoluminescence intensity between σ + and σ − excitation modulated at 10 (the black curve) and 100 kHz (the red curve), obtained by the locking-in technique in phase with σ + excitation. a.u., arbitrary unit. Full size image To provide useful physical insight into the key factors that can be tailored to optimize the DNP process, we performed a detailed rate equation analysis of P N as described in the Supplementary Methods . The results are partly displayed in Fig. 5 . As expected, τ A has a key role in the DNP efficiency. To build-up strong DNP, τ A should be shorter than ‘pure’ nuclear spin relaxation time ( τ N ), which causes nuclear spin leak. By decreasing τ A , a larger B N and stronger P N can be obtained. In combination with the measures to increase the efficiency of the spin-filtering/amplification effect, for example, by increasing electron capture coefficient γ e and/or the concentration of the spin-filtering defects ( N c ), complete nuclear spin polarization can be achieved at RT as shown in Fig. 5 . This is possible even when the initial spin polarization of conduction-band electrons generated by optical pumping is very low, for example, =5% as assumed in the simulations shown in Fig. 5 . 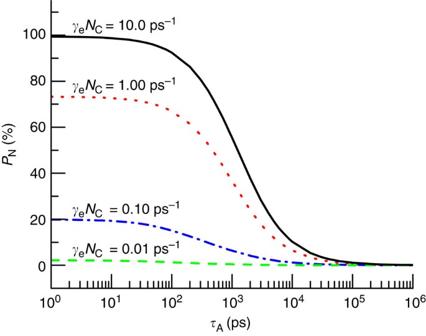Figure 5: Rate equation simulations of DNP. PNas a function ofτAandγeNc,simulated by the rate equation analysis. The key fitting parameters used are:τs=150 ps,τN=10 ns,τd=1 ns,T1SC=5 ns and=5%. Figure 5: Rate equation simulations of DNP. P N as a function of τ A and γ e N c, simulated by the rate equation analysis. The key fitting parameters used are: τ s =150 ps, τ N =10 ns, τ d =1 ns, T 1SC =5 ns and =5%. Full size image In summary, we demonstrated the realization of efficient, optically pumped DNP in a semiconductor at RT by a combined effect of SDR and HF coupling facilitated by the defect-engineered spin-filtering. We provided direct experimental evidence from ODMR that identifies the origin of the observed DNP as being due to nuclear spin hyperpolarization of the central Ga atom of the Ga i defect in GaNAs. We further showed that the observed DNP is very fast at RT, and can be completed within <5 μs. Though the RT DNP was demonstrated by optical pumping of conduction-band electrons, spin-polarized conduction-band electrons could also be provided by the alternative means of electrical spin injection. The physical principle of the DNP process is identical between the optical and electrical methods, apart from optical pumping versus electrical injection. The proposed new approach could thus pave a way to overcome a major obstacle in achieving strong DNP at RT, which could allow efficient and fast initialization, as well as computation if manipulation of nuclear spin qubits is to be carried out via e–n spin coupling. More significantly, it could enable these operations to be functional at RT that is highly desirable for practical applications of quantum computation using nuclear spin qubits. In terms of highly sensitive MRI, the impact of strong and efficient RT DNP is obvious as the sensitivity of MRI is directly linked to the degree of nuclear spin hyperpolarization. Our approach has an added advantage in enabling highly sensitive MRI agents to be prepared at RT in weak or even zero field. Samples The studied GaNAs samples were grown by gas-source or solid-source molecular beam epitaxy on (100)-oriented semi-insulating GaAs substrates with a 2,500 Å-thick GaAs buffer. Growth temperature was in the range of 390–500 °C. Nitrogen composition of the alloy ranges from 0.3 to 2.6%. Some of the samples were treated by post-growth rapid thermal annealing at 850 °C in N 2 ambient for 10 s. Experimental techniques Optical orientation experiments were performed at RT. Optical pumping above the bandgap energy of GaNAs was provided by circularly polarized light from a Ti:sapphire laser at a wavelength of 850–930 nm, propagating along the direction ( z ) normal to the sample surface (see Fig. 2a ). Circular polarization of excitation light was created by a waveplate, or an electrically controlled liquid crystal retarder, or an electro-optic modulator, in conjunction with a linear polarizer. In some cases, polarization of the excitation beam was modulated between different polarizations to facilitate applications of the lock-in amplifier technique either to increase signal-to-noise ratio or to register differential optical signals. Photoluminescence signals from the band-to-band optical transition were detected in a back scattering geometry by a cooled Ge-detector through a monochromator. ODMR measurements were performed under the optical orientation condition with a microwave frequency of 35.07 GHz. All measurements were done in the Faraday configuration, that is, with an external magnetic field applied along the z axis. To obtain strong DNP at RT, a high defect concentration and high optical excitation power are required. Both lead to acceleration of capture and recombination processes of conduction-band and defect electrons, which become extremely fast (<100 ps). This is much faster than the time response of photo-detectors available today for the concerned spectral range and microwave-induced spin transition rates, by more than three orders of magnitude, making ODMR signals too weak to be detectable at RT. Therefore, ODMR was performed at a low temperature (<50 K), when significant slow-down of carrier capture and recombination processes via the defects makes ODMR studies of DNP possible. Nevertheless the e–n spin flip-flops induced by the HF interaction, which leads to the observed DNP, should persist to RT as the process itself is expected to be insensitive to temperature. Physical principle of DNP driven by SDR and HF interaction For simplicity, we take as an example a simple e–n spin system with a single unpaired electron ( S =1/2) localized at a defect and a nuclear spin I =1/2 of the defect atom ( Fig.1a–d ). Four relative orientations between the electron and nuclear spins are possible, that is, ↑ , ↑ , ↓ and ↓ . Assuming that conduction-band electrons are completely spin polarized due to the spin-filtering effect, for example, spin-up under σ − optical excitation, the defect with a spin-up electron ( Fig. 1a ) will not capture a second electron due to the Pauli exclusion rule (that is, spin blockade). When the electron and nuclear spins are parallel, see Fig. 1a , the nuclear spin remains intact because the e–n spin flop-flop process driven by their Fermi-contact HF coupling with the operator is inactive (see below in the description of the spin Hamiltonian). For the ↑ spin configuration ( Fig. 1b ), on the contrary, the HF coupling can cause a mutual spin flip-flop between the electron and nucleus by the term . This leads to the ↓ configuration, which is equivalent to the case with an initial spin-down electron and spin-up nucleus shown in Fig.1c . Now, capture of a second electron with ↑ from the conduction-band by the defect becomes possible. This capture process is very efficient (<30 ps) refs 25 , 27 , making the reverse e–n spin flip-flop (that is, ↓ →↑ ) improbable. Once the defect is occupied by two spin-paired electrons, one of these two electrons can annihilate with a spin-unpolarized hole from the valence band. This will leave behind a localized electron that has a 50% chance of becoming spin-up. Repeated SDR processes as such will quickly convert the ↓ configuration ( Fig. 1c ) to the ↑ configuration ( Fig. 1a ), when both SDR and e–n spin flip-flops will cease to be active. In the fourth configuration (that is, ↓ shown in Fig. 1d ), the e–n spin flip-flip process driven by the operator is inactive. The SDR process will quickly drive ↓ to ↑ followed by the HF-induced e–n spin flip-flop that leads it to the ↓ configuration. As discussed above, SDR will finally drive it to the ↑ spin configuration. Therefore, the four possible spin configurations for the localized electron and nucleus will follow the paths illustrated by the dashed arrows shown in Fig. 1a–d and will all eventually end up with ↑ as the final and stable spin configuration. In other words, a combined effect of SDR and HF coupling can align both localized electron spin and nuclear spin towards the direction of the conduction-band electron spins generated by the spin-filtering effect, and will lead to strong spin polarization of both electron and nucleus at the defect. Spin hamiltonian The electron and nuclear spin levels of the Ga i defects with S =1/2 and I =3/2 can be described by the following spin Hamiltonian Here, the first and second terms are the electronic Zeeman and HF interaction, respectively. In the field range of our ODMR experiments, the first term is dominant. The nuclear Zeeman term is more than three orders of magnitude weaker than the electronic Zeeman term and can, therefore, be neglected here. is the Bohr magneton, g the g -factor of the electron localized at the defect and A the Fermi-contact HF parameter. The HF interaction , where the terms related to and have zero magnitude. Here, z refers to the quantization axis of the electron and nuclear spins that is defined along the direction of the external magnetic field. denotes the rising (+) or lowering (−) operators of the electron spin angular momentum, and is its counterpart for the nuclear spin. Ga has two stable isotopes, that is, 69 Ga and 71 Ga, each with a nuclear spin I =3/2. Therefore, two sets of four HF-split ODMR lines are expected for each Ga i defect. The intensity ratio between these two sets of the ODMR lines is governed by the ratio of natural abundance between the two isotopes, which is 60.4% for 69 Ga and 39.6% for 71 Ga. The HF splitting of 71 Ga should be 1.27 times larger than that of 69 Ga, reflecting the same difference in their nuclear magnetic moment. From a best fit of the spin Hamiltonian to the ODMR data shown in Fig. 3b , the g -factor and A parameter of the Ga i -D defect can be determined for the studied GaN 0.0036 As 0.9964 as g =2.01, A ( 69 Ga)=580.0 × 10 −4 cm −1 and A ( 71 Ga)=736.6 × 10 −4 cm −1 . These values slightly vary depending on the exact form of the Ga i interstitial defect, which can be modified under different growth conditions and post-growth treatments [25] , [30] . For the samples shown in Fig. 2 , the dominant spin-filtering defects in the GaN 0.026 As 0.974 epilayer are Ga i -A and Ga i -B, with A ( 69 Ga)=745 × 10 −4 cm −1 for Ga i -A and A ( 69 Ga)=1250 × 10 −4 cm −1 for Ga i -B. In the GaN 0.013 As 0.987 epilayer, on the other hand, the dominant spin-filtering defect is Ga i -C with A ( 69 Ga)=620 × 10 −4 cm −1 . How to cite this article: Puttisong, Y. et al . Efficient room-temperature nuclear spin hyperpolarization of a defect atom in a semiconductor. Nat. Commun. 4:1751 doi: 10.1038/ncomms2776 (2013).